In vitrofabrication of functional three-dimensional tissues with perfusable blood vessels Stem cell technology and tissue engineering have developed side by side and have the potential to lead to regenerative therapies for the treatment of many patients suffering from various diseases. As Langer and Vacanti reported the fabrication of cartilage tissue in the shape of an ear by seeding cell suspensions onto a three-dimensional (3-D) biodegradable polymer scaffold, scaffold-based tissue engineering has rapidly spread around the world [1] , [2] , [3] . This technology has already been used for several clinical applications of bioengineered tissues, including bone, cartilage, skin and large blood vessels [4] , [5] , [6] . On the other hand, we have developed cell-sheet-based tissue engineering, which utilizes two-dimensional (2-D) contiguous monolayer cells in a cell sheet collected from a temperature-responsive culture surface [7] , [8] . The cell sheet is easily transferred onto damaged organs and 3-D tissues are bioengineered simply by stacking the 2-D cell sheets. Clinical applications to date include oral mucosal epithelial cell sheets transplanted to repair damage from cornea and oesophagus diseases, and myoblast sheets have been implanted to treat severe heart failure [9] , [10] , [11] . Furthermore, synchronously pulsatile myocardial tissues have been successfully fabricated by stacking rat cardiac cell sheets [12] . Both of these technologies have realized native tissue-like 3-D structures; however a long-standing critical obstacle in tissue engineering is the formation of perfusable blood vessels in vitro for oxygen and nutrient supply, and waste removal. Usually, in vivo host-originated blood vessel formation is to be expected, but primary ischaemia before sufficient neovascularization limits the viability and thickness of engineered tissue [13] . In vitro endothelial cell (EC) coculture has been a recent focus and reported to enhance in vivo vascular formation. However, the effectiveness is limited by the immature structure of in vitro cultured ECs, because they only produce EC networks with a partial tubular structure. After all, the thickness of viable tissue is limited by the time period for in vivo vascular maturation and connexion with the host blood vessels. Therefore, new techniques for in vitro formation of mature blood vessels with continuous media-perfusable lumens is critical for the future development of tissue engineering. Here we demonstrate a technology for in vitro fabrication of functional 3-D tissues with perfusable blood vessels. In vitro engineered tissue survived after transplantation by successfully connecting to the host blood vessels. Vascular bed preparation in a perfusion bioreactor system To mimic in vivo conditions, cardiac cell sheets cocultured with ECs were transferred onto a vascular bed using a resected section of femoral tissue containing a connectable artery and vein, which was then perfused with culture medium in vitro . We hypothesized that the cocultured ECs could form new blood vessels that would connect with the blood vessels originating from the vascular bed, so that media supplied through these newly formed vessels would allow the cell sheet constructs to survive ( Fig. 1a ). 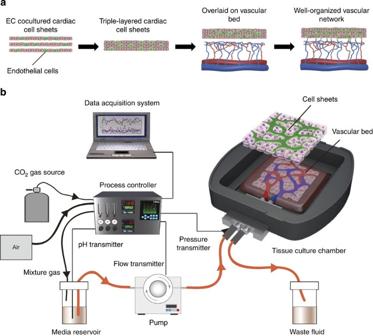Figure 1:In vitroengineering of functional 3-D tissue with perfusable blood vessels. (a) To engineer cell sheet constructs with perfusable blood vessels, EC cocultured cardiac cell sheets are stacked, and then overlaid on a vascular bedin vitro. After appropriate perfusion using a bioreactor, the cocultured ECs formed new blood vessels and connected with the blood vessels that originated from the vascular bed. Finally, the cell sheet constructs survive via the media supplied through the new vessels that formedin vitro. (b) The engineered constructs are perfused in a custom-made bioreactor. The bioreactor is a one-pass system consisting of a delivery pump, a custom-made tissue culture chamber, pH transmitter, flow transmitter, pressure transmitter, CO2gas source, process controller and data acquisition system. The construct is placed in the tissue culture chamber to become a vascular bed and the femoral vessels are connected to two micro polyurethane tubes for culture media perfusion. The flow is generated by a delivery pump from the media reservoir monitored by a pressure sensor positioned on the arterial inlet side, passing through the tissue culture chamber to exit into a waste fluid tank. The pH is measured and controlled via a process controller to verifying the concentration of CO2gas. The pH, temperature and arterial pressure sensors are connected to the computer via a process controller. Figure 1: In vitro engineering of functional 3-D tissue with perfusable blood vessels. ( a ) To engineer cell sheet constructs with perfusable blood vessels, EC cocultured cardiac cell sheets are stacked, and then overlaid on a vascular bed in vitro . After appropriate perfusion using a bioreactor, the cocultured ECs formed new blood vessels and connected with the blood vessels that originated from the vascular bed. Finally, the cell sheet constructs survive via the media supplied through the new vessels that formed in vitro . ( b ) The engineered constructs are perfused in a custom-made bioreactor. The bioreactor is a one-pass system consisting of a delivery pump, a custom-made tissue culture chamber, pH transmitter, flow transmitter, pressure transmitter, CO 2 gas source, process controller and data acquisition system. The construct is placed in the tissue culture chamber to become a vascular bed and the femoral vessels are connected to two micro polyurethane tubes for culture media perfusion. The flow is generated by a delivery pump from the media reservoir monitored by a pressure sensor positioned on the arterial inlet side, passing through the tissue culture chamber to exit into a waste fluid tank. The pH is measured and controlled via a process controller to verifying the concentration of CO 2 gas. The pH, temperature and arterial pressure sensors are connected to the computer via a process controller. Full size image To obtain a vascular bed with a complete arterio-venous (AV) loop, rat femoral muscle tissue, including branches of the femoral artery and vein, was partially resected from the surrounding tissues and peripheral blood vessels. The tissue with the artery and vein was then immediately returned to its original position and incubated in the host body for 1 week. After remodelling of the tissue and blood vessel networks, the whole construct, including the femoral artery and vein, was resected from the rat. Then, the construct was placed in a tissue culture chamber to become a vascular bed and the femoral vessels were connected to two thin polyurethane tubes for the culture media perfusion ( Fig. 1b ). The vascular bed was perfused with culture media, which included 6% fetal bovine serum from the inlet tube connecting to the femoral artery. The media pH (7.4) and perfusion rate (50 μl min −1 ) were maintained in a steady state by gas and pump controllers, respectively. In addition, the inlet pressure (49±26 mmHg) and the outlet waste media volume (47±15% of perfused media) were continuously monitored. Although significant volume of the media exuded from the tissue surface, it is a natural phenomenon as observed with in vivo intestinal fluids, which are usually returned to vein or lymph vessels under closed conditions. Using this bioreactor system, the tissues, including the AV networks were continuously perfused as a vascular bed. Tight connection of cardiac cell sheets on the vascular bed Next, neonatal rat cardiac cells, with or without ECs, were cultured on temperature-responsive culture dishes. After a 4-day culture, confluent cells were harvested as 2-D contiguous cell sheets from the dishes only by lowering the temperature. As previously reported, cocultured cell sheets maintained their prevascular EC networks [14] , [15] . Three cell sheets were stacked together, and then the triple-layered tissue was overlaid on the vascular bed in the bioreactor system; because three layers is the thickness limit for layered cell sheets without blood vessels. Biological extracellular proteins remain underneath the cell sheets, even after detachment from the culture dishes, and this realized a tight and rapid adhesion not only between each cell sheet, but also between the cell sheet and the vascular bed [16] . Therefore, these tightly connected tissues were able to be continuously cultivated in vitro without any delamination. In vitro perfusable blood vessel formation By using this bioengineered tissue culture system, we compared the perfusable blood vessel formation among four groups (each n =4), with and without EC coculture, and with or without the addition of fibroblast growth factor 2 (FGF-2) in the perfusion media. FGF-2 is well-known as an accelerator of neovascularization [17] . After a 3-day culture, black ink was perfused through the constructs and fixed for histological analyses. Haematoxilin and eosin (HE) staining of black ink-perfused tissues demonstrated that there was no luminal structure nor any ink detected within the cell sheet layers in the non-coculture groups, regardless of FGF-2 administration ( Fig. 2a ). In the case of cocultured constructs without FGF-2 perfusion, significant tubular structure was observed within the constructs; however, there was hardly any ink detected within the structure ( Fig. 2c ). On the other hand, in the case of FGF-2-treated, cocultured constructs, the black ink reached well within the tubular structure of the cell sheet layers and perfused throughout the constructs ( Fig. 2d ). The infused black ink was thoroughly perfused and successfully returned to the outlet. EC staining also revealed that there was no blood vessel structure within the non-cocultured cardiac tissues ( Fig. 2e ), but that many tubular blood vessel structures were formed within the cardiac tissues cocultured with ECs ( Fig. 2g ). These data confirmed that cocultured ECs contribute to blood vessel tubular structure formation within the cell sheet constructs, and that FGF-2 promotes perfusable blood vessel communication between the constructs and the vascular bed. 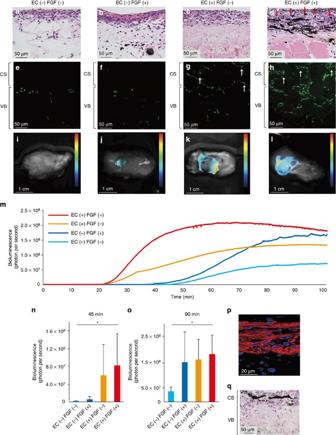Figure 2: Perfusable blood vessel formation and viable cardiac tissue fabrication. Blood vessel formation and tissue viability were evaluated among the four groups, with and without EC coculture, and with or without FGF-2 administration in the perfusion medium. Each group was indicated as EC (−) FGF (−), EC (−) FGF (+), EC (+) FGF (−) and EC (+) FGF (+). (a–d) HE staining after a 3-day perfusion culture. Neither a luminal structure nor perfused black ink were detected in either the EC (−) FGF (−) group or in the EC (−) FGF (+) group. In the EC (+) FGF (−) group, a luminal structure was observed, but the black ink was hardly detected within it. In the EC (+) FGF (+) group, the infused black ink thoroughly reached the blood vessel structure within cell sheet layers (red arrows). (e–h) CD31 staining for ECs. No blood vessel structure was observed within the cell sheet layers in either the EC (−) FGF (−) group or the EC (−) FGF (+) group. Significant tubular blood vessel structures (white arrows) were observed in the EC (+) FGF (−) group and in the EC (+) FGF (+) group. cell sheet (CS) indicates cell sheet constructs and vascular bed (VB) indicates vascular beds. (i–o) Luciferase-expressing triple-layer cell sheets were overlaid on the vascular beds. After continuous luciferin infusion, serial bioluminescent imaging of each group was analysed. The images captured at 45 min are shown (i–l). Representative dynamic tracing is demonstrated (m). The bioluminescent intensity at 45 and 90 min is shown (n,o). The intensity increased in the early phase in the EC (+) FGF (−) group and the EC (+) FGF (+) group. On the other hand, it increased in the late phase in the EC (−) FGF (−) group and the EC (−) FGF (+) group. FGF-2 accelerated the increasing rate, regardless of EC coculture. Data are shown as mean±s.d. (*P<0.05) (n=4). (p) Sarcomeric α-actinin staining (red) with nuclei staining (blue) revealed well-differentiated sarcomeres within the cell sheet construct in the EC (+) FGF (+) group. (q) HE staining showed that perfused black ink is occasionally detected EC(+) FGF(−) group. Figure 2: Perfusable blood vessel formation and viable cardiac tissue fabrication. Blood vessel formation and tissue viability were evaluated among the four groups, with and without EC coculture, and with or without FGF-2 administration in the perfusion medium. Each group was indicated as EC (−) FGF (−), EC (−) FGF (+), EC (+) FGF (−) and EC (+) FGF (+). ( a – d ) HE staining after a 3-day perfusion culture. Neither a luminal structure nor perfused black ink were detected in either the EC (−) FGF (−) group or in the EC (−) FGF (+) group. In the EC (+) FGF (−) group, a luminal structure was observed, but the black ink was hardly detected within it. In the EC (+) FGF (+) group, the infused black ink thoroughly reached the blood vessel structure within cell sheet layers (red arrows). ( e – h ) CD31 staining for ECs. No blood vessel structure was observed within the cell sheet layers in either the EC (−) FGF (−) group or the EC (−) FGF (+) group. Significant tubular blood vessel structures (white arrows) were observed in the EC (+) FGF (−) group and in the EC (+) FGF (+) group. cell sheet (CS) indicates cell sheet constructs and vascular bed (VB) indicates vascular beds. ( i – o ) Luciferase-expressing triple-layer cell sheets were overlaid on the vascular beds. After continuous luciferin infusion, serial bioluminescent imaging of each group was analysed. The images captured at 45 min are shown ( i – l ). Representative dynamic tracing is demonstrated ( m ). The bioluminescent intensity at 45 and 90 min is shown ( n , o ). The intensity increased in the early phase in the EC (+) FGF (−) group and the EC (+) FGF (+) group. On the other hand, it increased in the late phase in the EC (−) FGF (−) group and the EC (−) FGF (+) group. FGF-2 accelerated the increasing rate, regardless of EC coculture. Data are shown as mean±s.d. (* P <0.05) ( n =4). ( p ) Sarcomeric α-actinin staining (red) with nuclei staining (blue) revealed well-differentiated sarcomeres within the cell sheet construct in the EC (+) FGF (+) group. ( q ) HE staining showed that perfused black ink is occasionally detected EC(+) FGF(−) group. Full size image Cell sheet survival via functional blood vessels We also examined the media supply to cell sheet layers and their viability among the same four groups (each n =4) using a luciferin-luciferase bioluminescent imaging system. Cocultured or non-cocultured cardiac cell sheets were fabricated from luciferase-transgenic rat hearts, and triple-layer constructs were overlaid on the vascular bed in the bioreactor system. After a 3-day perfusion culture, with or without FGF-2 administration, luciferin was continuously infused from the artery side and when it reached the cell sheets it promptly displayed luminescence. The early bioluminescence increasing state indicated that the media supply process includes both direct media perfusion via the blood vessel structure and media diffusion through the tissues. On the other hand, the late plateau state represented the total viability of the survived cardiac tissues. Captured bioluminescent images showed an earlier start of signals and higher signals at 45 min after luciferin infusion in the two groups with EC coculture compared with the two groups without coculture ( Fig. 2i–n ; Supplementary Movie 1 ). This indicated that luciferin directly reached the constructs via the blood vessel structure in the coculture cases, whereas luciferin diffused from the blood vessels of the vascular bed and slowly reached the tissues in the non-coculture cases. Furthermore, the increasing rate was steeper in the FGF-2-treated case than in the non-treated case ( Fig. 2m ). Consistent with the histological analyses, FGF-2 accelerated functional communications between the newly formed capillaries within the cocultured tissues and the pre-existing blood vessels within the vascular bed, leading to faster media perfusion. In the non-coculture cases, cultivation with FGF-2 also tended to initiate a faster increase of the signals than that without FGF-2, so that the final tissue viability was comparative with the cocultured constructs. It was considered that FGF-2 might have an effect on the blood vessel structure within the vascular bed and promote media diffusion from the bed to the non-vascularized cell sheet layers, supporting the survival of triple-layer constructs, which are at the limit of thickness without blood vessels. Statistically, FGF-2-treated, cocultured constructs showed significantly higher signals both at 45 and 90 min, compared with the non-FGF-2-treated, non-cocultured constructs ( Fig. 2n ). These morphological and luciferin infusion analyses confirmed that the combination of EC coculture and FGF-2 perfusion culture realized in vitro perfusable blood vessel formation, which contributes to the in vitro survival of 3-D tissues. Furthermore, the media-perfused cardiac tissues presented synchronous pulsation in vitro ( Supplementary Movie 2 ), as well as the characteristic morphology of native heart tissue, including well-differentiated sarcomeres ( Fig. 2p ). Contribution of ECs to blood vessel formation Next we examined the contribution of cocultured ECs by using green fluorescence protein (GFP)-expressing ECs. Scanning 2-D fluorescent images were obtained after the cocultured constructs were finally perfused with red fluorescent dextran ( Fig. 3a ). Without FGF-2 treatment, GFP-positive EC networks were maintained within the cell sheets, but dextran was hardly observed in the cell sheets ( Fig. 3b–d ; Supplementary Movie 3 ). By contrast, FGF-2 treatment allowed significant red fluorescent dextran to pass through the GFP-positive EC tubular structures ( Fig. 3e–g ; Supplementary Movie 4 ). In another experiment, we perfused 4-μm-diameter red fluorescent spheres which similarly revealed many of the microspheres in the GFP-positive blood vessels of the FGF-2-treated constructs ( Fig. 3h–j ; Supplementary Movie 5 ). Furthermore, in the FGF-2-treated case, cross-sectional fluorescent images, which can differentiate between blood vessels that originated from both the cell sheet and the vascular bed, clearly shows migration of cocultured GFP-positive ECs into the vascular bed and directly communicating chimerical blood vessels ( Fig. 3k ). By contrast, when the GFP-negative cell sheet layers were overlaid on a GFP-expressing vascular bed, GFP-positive cells hardly migrated into the cell sheet constructs ( Fig. 3m ). These data indicated that prevascular endothelial networks migrate into the vascular bed and connect to the blood vessels originating from the bed, leading to the formation of functional tubular blood vessels in the culture chamber when using FGF-2-containing media, similar to that found in vivo . 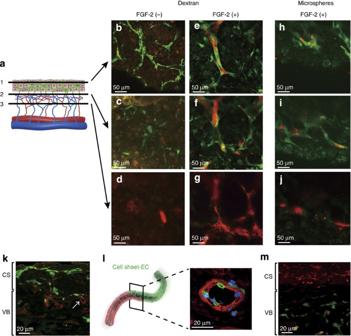Figure 3: Contribution of cocultured ECs within the construct. (a) Scanning two-dimensional fluorescent images of the constructs containing cocultured green fluorescence protein (GFP)-expressing ECs were obtained after the constructs were perfused with red fluorescent dextran. Three xy images at different depths of the cell sheet (CS) regions (b,eandh), border region (c,fandi) and vascular bed (VB) region (d,gandj) are presented. (b–d) Without FGF-2 treatment, the GFP-positive EC networks remain within the cell sheets, but dextran is hardly observed within the cell sheets. (e–g) In the case of FGF-2-treated constructs, red fluorescent dextran passed through the GFP-positive EC tubular structures. (h–j) When 4-μm-diameter red fluorescent spheres were perfused, many microspheres were observed in the GFP-positive blood vessels of the cell sheets when treated with FGF-2. (k) Immunostaining with CD31 (red: all ECs) and GFP (green: ECs originated from the cell sheet) demonstrated that cocultured ECs migrated into the vascular bed and connected to the blood vessels within the bed. An arrow indicates the communication between migrating ECs originated from the cell sheet and vascular bed originated ECs. (l) Fused blood vessels containing both vascular bed (red) and cell sheet (green)-derived ECs were present in the vascular bed. (m) By contrast, when GFP-negative cell sheets were overlaid on the GFP-expressing vascular bed, GFP-positive cells never migrated into the cell sheet layers. Figure 3: Contribution of cocultured ECs within the construct. ( a ) Scanning two-dimensional fluorescent images of the constructs containing cocultured green fluorescence protein (GFP)-expressing ECs were obtained after the constructs were perfused with red fluorescent dextran. Three xy images at different depths of the cell sheet (CS) regions ( b , e and h ), border region ( c , f and i ) and vascular bed (VB) region ( d , g and j ) are presented. ( b – d ) Without FGF-2 treatment, the GFP-positive EC networks remain within the cell sheets, but dextran is hardly observed within the cell sheets. ( e – g ) In the case of FGF-2-treated constructs, red fluorescent dextran passed through the GFP-positive EC tubular structures. ( h – j ) When 4-μm-diameter red fluorescent spheres were perfused, many microspheres were observed in the GFP-positive blood vessels of the cell sheets when treated with FGF-2. ( k ) Immunostaining with CD31 (red: all ECs) and GFP (green: ECs originated from the cell sheet) demonstrated that cocultured ECs migrated into the vascular bed and connected to the blood vessels within the bed. An arrow indicates the communication between migrating ECs originated from the cell sheet and vascular bed originated ECs. ( l ) Fused blood vessels containing both vascular bed (red) and cell sheet (green)-derived ECs were present in the vascular bed. ( m ) By contrast, when GFP-negative cell sheets were overlaid on the GFP-expressing vascular bed, GFP-positive cells never migrated into the cell sheet layers. Full size image In vitro scaling-up of the 3-D vascularized tissue To scale-up production of bioengineered tissues, we have already demonstrated one possible solution in vivo . Multiple transplantation of triple-layer cell sheets produced thicker tissues under in vivo conditions [18] . Therefore, to scale-up in vitro , triple-layer cocultured cardiac cell sheets could be repeatedly overlaid on the vascular bed and perfused using the bioreactor system. A second triple-layer tissue was overlaid on the first graft after 3 days cultivation and the whole construct was perfused for a further 3 days ( Fig. 4a ). By comparison, a six-layer cell sheet tissue was overlaid on the vascular bed and cultured for 6 days ( Fig. 4b ). Although blood cells perfused at the end of the cultivation were able to reach the cardiac tissues in both procedures, the two-step procedure produced thicker and more cell-dense cardiac tissues than the single-step six-layer procedure ( Fig. 4c–f ). Some cells became necrotic in the single-step six-layer procedure, because of the primary diffusion limit of oxygen and nutrition and waste accumulation within the six-layer tissues. On the other hand, allowing time for functional neovascularization within the first triple-layer tissue produces a sufficient vascular bed for the second triple-layer, so that the final six-layer tissue was totally vascularized without any necrosis. Bioluminescent imaging analyses using luciferase-expressing cell sheets also clearly demonstrated greater tissue survival in the two-step procedure than in the single-step procedure ( n =4, Fig. 4g–i ; Supplementary Movie 6 ). A thick 12-layer construct is produced by overlaying triple-layer cell sheets four times on a vascular bed ( Fig. 4j ). This successful procedure has opened up a new possibility for scaling-up the production of bioengineered tissues in vitro . 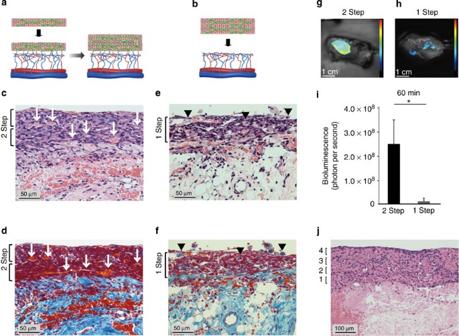Figure 4: Double-step overlaying of triple-layer cell sheets and viability assay. (a) The double-step overlaying is schematically illustrated. Triple-layer cocultured cardiac cell sheets are overlaid on the vascular bed and perfused. After 3 days of cultivation, to provide sufficient vascularization within the first graft, the second triple-layer tissue is overlaid on the first graft and the construct is perfused for a further 3 days. Finally, the whole construct is thoroughly vascularized. (b) The single-step overlaying with six-layer cell sheets is schematically illustrated. Six-layer cell sheet tissues are overlaid, in one step, on the vascular bed and perfused for 6 days. (c,d) HE and Azan staining for blood-perfused double-step constructs showed that blood cells well reached the six-layer cell sheets (white arrows) and that thicker and more cell-dense tissue was successfully fabricated. (e,f) HE and Azan staining for blood cell-perfused one-step constructs shows some necrotic cells (black arrow heads) and relatively cell-sparse tissues. (g–i) After continuous luciferin infusion, serial bioluminescent imaging of each group was analysed. The images captured at 60 min are shown (g,h). The intensity from the double-step procedure was significantly higher than that from the single-step procedure (i). Data are shown as mean±s.d. (*P<0.05) (n=4). Triple-layer cell sheets are overlaid four times on the vascular bed to produce a thick 12-layer construct (j). Figure 4: Double-step overlaying of triple-layer cell sheets and viability assay. ( a ) The double-step overlaying is schematically illustrated. Triple-layer cocultured cardiac cell sheets are overlaid on the vascular bed and perfused. After 3 days of cultivation, to provide sufficient vascularization within the first graft, the second triple-layer tissue is overlaid on the first graft and the construct is perfused for a further 3 days. Finally, the whole construct is thoroughly vascularized. ( b ) The single-step overlaying with six-layer cell sheets is schematically illustrated. Six-layer cell sheet tissues are overlaid, in one step, on the vascular bed and perfused for 6 days. ( c , d ) HE and Azan staining for blood-perfused double-step constructs showed that blood cells well reached the six-layer cell sheets (white arrows) and that thicker and more cell-dense tissue was successfully fabricated. ( e , f ) HE and Azan staining for blood cell-perfused one-step constructs shows some necrotic cells (black arrow heads) and relatively cell-sparse tissues. ( g – i ) After continuous luciferin infusion, serial bioluminescent imaging of each group was analysed. The images captured at 60 min are shown ( g , h ). The intensity from the double-step procedure was significantly higher than that from the single-step procedure ( i ). Data are shown as mean±s.d. (* P <0.05) ( n =4). Triple-layer cell sheets are overlaid four times on the vascular bed to produce a thick 12-layer construct ( j ). Full size image In vivo survival of beating cardiac tissues Our next step was to transplant in vitro bioengineered vascularized tissue in vivo . The six-layer tissue graft, engineered by the double-step overlaying of triple-layer luciferase-expressing cell sheets, was removed from the bioreactor system after a 6-day cultivation, and transplanted in the neck of a nude rat. The protruding femoral artery and vein of the graft were then reconnected to the carotid artery and the jugular vein, respectively, by a cuff technique as previously reported ( Fig. 5a ); [19] . By comparison, six-layer grafts with vascular beds were transplanted without vessel anastomoses ( Fig. 5b ), and also six-layer cell sheets without a vascular bed were simply transplanted ( Fig. 5c ). In vivo imaging of bioluminescence revealed the highest viability in cases of grafting via blood vessel anastomoses ( Fig. 5d–g , n =4). On the other hand, the viabilities were very low in both the grafts without vessel anastomoses and in the simple six-layer constructs without a vascular bed, indicating that tissue necrosis was due to primary ischaemia ( Fig. 5e–g ). The vascularized graft with blood vessel anastomoses also maintained its vascular structure and beating for 2 weeks after the procedure ( Fig. 5h ). It showed the uniform distribution of ECs and the characteristics of a micro blood vessel ( Fig. 5i ). This successful grafting demonstrated the clinical potential of transplanting in vitro bioengineered tissues with connectable and functional AV networks. 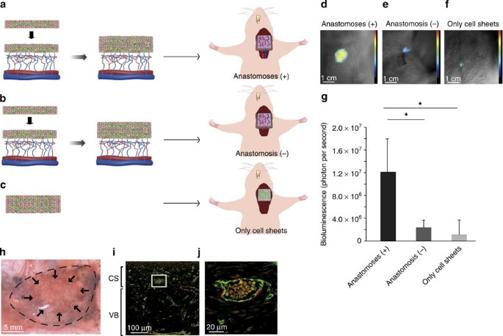Figure 5: Transplantation ofin vitrovascularized cardiac tissues. (a) The six-layer tissue graft engineered by the double-step procedure was removed from the bioreactor system and transplanted in the neck of a nude rat with anastomosis between the protruding femoral vessels of the graft and the connectable neck blood vessels of the host rat. (b) The six-layer graft was transplanted without the vessel anastomosis. (c) The six-layer cell sheets (CS) without the vascular bed (VB) were simply transplanted. (d–f)In vivobioluminescent imaging of each graft is shown. Obvious signals were observed in the graft with vessel anastomoses (d). The intensity was low in the graft without anastomosis (e) and in the graft without a vascular bed (f). (g) The intensity was significantly the highest in the graft with vessel anastomosis, compared with the other two grafts. Data are shown as mean±s.d. (*P<0.05) (n=4). (h) The vascularized graft with blood vessel anastomoses also maintained its vascular structure at 2 weeks after the procedure. Dotted line indicates the area of the graft with the vascular bed and arrows indicate the area of the cell sheet layers. (i) Immunostaining for CD31 (green: ECs) and calponin (red: smooth muscle cell) shows the uniform distribution of micro blood vessels in the cell sheet construct. (j) The detail in the white box ofiillustrates the characteristics of a matured blood vessels including red blood cells. Figure 5: Transplantation of in vitro vascularized cardiac tissues. ( a ) The six-layer tissue graft engineered by the double-step procedure was removed from the bioreactor system and transplanted in the neck of a nude rat with anastomosis between the protruding femoral vessels of the graft and the connectable neck blood vessels of the host rat. ( b ) The six-layer graft was transplanted without the vessel anastomosis. ( c ) The six-layer cell sheets (CS) without the vascular bed (VB) were simply transplanted. ( d – f ) In vivo bioluminescent imaging of each graft is shown. Obvious signals were observed in the graft with vessel anastomoses ( d ). The intensity was low in the graft without anastomosis ( e ) and in the graft without a vascular bed ( f ). ( g ) The intensity was significantly the highest in the graft with vessel anastomosis, compared with the other two grafts. Data are shown as mean±s.d. (* P <0.05) ( n =4). ( h ) The vascularized graft with blood vessel anastomoses also maintained its vascular structure at 2 weeks after the procedure. Dotted line indicates the area of the graft with the vascular bed and arrows indicate the area of the cell sheet layers. ( i ) Immunostaining for CD31 (green: ECs) and calponin (red: smooth muscle cell) shows the uniform distribution of micro blood vessels in the cell sheet construct. ( j ) The detail in the white box of i illustrates the characteristics of a matured blood vessels including red blood cells. Full size image Here we have fabricated functional 3-D cardiac tissues in vitro with perfusable vascular networks using cell-sheet-based tissue engineering and a novel bioreactor system. The advantage of cell sheet technology is the direct cell-to-cell communications between cell sheets and between a cell sheet and a host tissue, which initiate electrical communications and vascular network formation within the engineered tissues. Various types of extracellular matrix and membrane proteins, including fibronectin and integrin, are preserved underneath the cell sheets and act as adhesive agents when cell sheets are stacked on each other or transferred onto other tissues [20] . Cardiac cell sheets communicate electrically within 30 min via fast gap junction formation, and the EC networks within cell sheets also communicate between cell sheets [21] , [22] , [23] . In this study, the cocultured ECs and the direct attachment of the cell sheet onto the vascular bed might have initiated the formation of the functional vascular network between the cell sheets and the vascular bed. The experiments using GFP-expressing cells clearly revealed that cocultured ECs within cell sheets migrated into the vascular bed and connected to its blood vessels. In addition, media perfusion through the blood vessels in the vascular bed probably triggered the tubular structure formation in the EC network of the cell sheets, just as observed after in vivo cell sheet transplantation. Several studies have reported the possibility of in vitro functional blood vessel formation, however, completely perfusable blood vessel formation within cell-dense tissues has not been reported [24] , [25] , [26] , [27] . Although preformed 3-D scaffolds, including microcapillary lumens, may realize a native tissue-like structure, high-density cell seeding is difficult and leaky blood vessels are problematic. We believe that trying to mimic the natural regenerative growth in organs is a better approach to tissue engineering. Therefore, the simultaneous reconstruction of tissues together with their own blood vessels may be more appropriate for cell-dense tissue fabrication. From this point of view, the present step-by-step procedure based on cell sheet stacking technology seems to be feasible for in vitro fabrication of viable tissues with an appropriate vascular network formation that can be scaled up. In this study, serial bioluminescent imaging contributed to important information about media supply dynamics, in addition to tissue viability. Regarding in vivo imaging, luminescent intensity increased faster and the peak came earlier in luciferin infused via blood vessels than through intraperitoneal infusion. This indicates that the direct supply of luciferin through blood vessels initiates a rapid response, but that gradual diffusion through the tissues causes a delayed response [28] . Similarly, the present data revealed an earlier start of bioluminescent intensity in the cocultured constructs than in the non-cocultured constructs, and therefore we considered that perfusable blood vessel communications had developed between the cell sheet construct and the vascular bed. In contrast to the black ink perfusion throughout the FGF-treated, cocultured constructs, the ink was hardly detected in most cross-sections of the non-FGF-2-treated, cocultured constructs ( Fig. 2c ), and only partial perfusion was occasionally observed in some sections ( Fig. 2q ). Therefore, the numerous blood vessel connexions due to FGF-2 treatment might have contributed to the rapid media flow through newly formed blood vessels and the early and fast increase in luminescence. On the other hand, partial blood vessel communications in the non-FGF-2-treated constructs might have caused stagnant media flow in the blood vessel structure, leading to the early but slow increase of signals. We have repeated the procedure up to four times and successfully fabricated a 12-layer construct ( Fig. 4j ), however, the thickness does not increase linearly in accordance with the number of layered cell sheets. When multi-step procedures are performed with the same cultivation conditions, uniform perfusion may be insufficient for whole-tissue survival, resulting in a reduction in the thickness of the final tissue. It seems that at least the flow rate should be increased in accordance with tissue mass to increase the thickness. Moreover, the periods required for sufficient neovascularization within the first triple-layer cell sheets in vivo and in vitro are 1 and 3 days, respectively. This significant gap is considered to be caused by the differences in the composition of the liquids perfused, blood vessel pressure and surrounding atmosphere conditions. Therefore, further biological and mechanical optimization should also accelerate vascular formation and improve the efficiency of scaling-up. In this study, 3-D pulsatile cardiac tissues including a completely perfusable AV loop were developed. By using a native vascular bed with surgically connectable artery and vein, in vitro bioengineered vascularized tissues were retransplanted with blood vessel anastomoses and survived in vivo . In clinical applications, candidates for vascular beds could include an antero lateral thigh flap with the descending branches of the lateral circumflex femoral artery and vein, or a serratus flap with the branches of the dorsal thoracic artery and vein. For engineering large-scale cardiac tissues, cardiomyocytes differentiated from embryonic stem and induced pluripotent stem cells may be future possible cell sources. We have already established the technology for expanding human induced pluripotent stem cell-derived cardiomyocytes and have successfully made cell sheets with them [29] . The size and shape of cell sheets can also be controlled by culture surface modification. Future optimization of human resectable tissues including a thick artery and vein, a human implantable cardiac cell source and perfusion culture conditions may allow in vitro fabrication of clinically transplantable large-scale tissue. These constructs are also useful for basic biology and drug screening as in vitro models. The connectable artery and vein is helpful for drug administration into tissues, which can mimic in vivo conditions and may be an alternative to animal experiments. In conclusion, we have shown that the in vitro construction of perfusable blood vessel within viable cell-dense tissues is possible, that these are suitable for subsequent transplantation and that their production can be scaled up. This technique for in vitro tissue engineering may be applied to many other tissue types than the cardiac tissue demonstrated here, and may facilitate the discovery of new biological and medical insights, as well as lead to further advances in tissue engineering and its potential therapeutic application. All animal experiments were performed according to the ‘Guidelines of Tokyo Women’s Medical University on Animal Use’. Vascular bed fabrication An engineered vascular bed to promote angiogenesis was made from rat femoral muscle, which included an artery and vein. Fischer 344 athymic rats (250–350 g, male, Charles River Japan, Tokyo, Japan) and GFP-expressing Sprague-Dawley (SD) neonatal rats (SD-TgN [Act-EGFP] OsbCZ-004, SLC, Hamamatsu, Japan) were anesthetized with 2% inhaled isoflurane. The rat femoral muscle tissue was partially resected from the surrounding tissue and peripheral blood vessels by using a thermal cautery unit (TCU-150, Bio Research Center, Nagoya, Japan). The tissue including the artery and vein was reset to the original position. One week after the incubation in the host body, the whole construct was resected together with the femoral artery and vein under anaesthesia and heparinization (400 IU kg −1 , intravenous injection). The blood in the construct was washed out with lactated ringer’s solution. Rats were then euthanized with overdoses of pentobarbital. Bioreactor set-up and tissue perfusion culture The bioreactor is a one-pass system consisting of a microprocessor-controlled delivery pump (IPC-N, ISMATEC, Germany), a custom-made tissue culture chamber (Tokai Hit, Shizuoka, Japan), a pH probe (ABLE, Tokyo, Japan), a dissolved oxygen probe (ABLE), a pH transmitter (ABLE), flow transmitter (ABLE), a pressure transmitter (Edwards Lifesciences, Tokyo, Japan), CO 2 gas flow controllers and a data acquisition system (ABLE). A glove box was used to maintain a temperature of 37 °C (AS ONE, Tokyo, Japan). The tubing used for connexions was Micro-Renathane (I.D. 0.3 and 0.6 mm, Bio Research Center) and the pump tubing was Pharmed Ismaprene (I.D. 1.3 mm, ISMATEC). The pH conditions were measured and controlled via a process controller to verify the concentration of CO 2 gas in the media reservoir. The outlet waste media volumes were measured by electrical balance (A&D, Tokyo, Japan). The vascular bed was placed in a tissue culture chamber and perfused with culture media including 6% fetal bovine serum at 50 μl min −1 by the delivery pump through the inlet tube connected to the femoral artery. The data of pH, temperature, arterial pressure and perfused media volume were recorded during the cultivation. For enhancement of neovascularization, 16 ng ml −1 rat FGF-2 (PeproTech, Rocky Hill, NJ) was added into the culture media. Cell sheet fabrication Cardiac cells were isolated from the ventricles of 1-day-old SD neonatal rats (SLC), GFP-positive SD neonatal rats (SLC) and firefly luciferase-expressing Lewis neonatal rats (LEW-Tg [Rosa-luc] 11 jmsk) according to previously described procedures [11] . Endothelial cells (ECs) were separated from primary myocardial cell suspensions by magnetic cell sorting (Miltenyi Biotech GmbH, Bergisch Gladbach, Germany) using mouse monoclonal anti-rat CD31 antibody (MCA1334G, Serotec Ltd., Oxford, UK), as previously described [13] . To fabricate cocultured cardiac cell sheets, GFP-negative cardiac cells without ECs and purified GFP-positive ECs were mixed at a ratio of 4:1, and were cultured at a density of 2.4 × 10 6 cells on 35-mm temperature-responsive culture dishes (CellSeed, Inc., Tokyo, Japan) at 37 °C in a humidified atmosphere containing 5% CO 2 . After 4 days, the cocultured cardiac cells were transferred to another incubator set at 20 °C for 1 h, to release the cultured cells as intact sheets. Stacking and transfer to the vascular bed The cardiac cell sheets, which detached spontaneously from temperature-responsive culture dishes, were suspended in the aqueous media. To layer the cell sheets, one cell sheet with culture media was gently aspirated into the tip of a pipette and transferred onto a new temperature-responsive culture dish. After dropping culture media to smoothly spread the cell sheets, the dishes were incubated at 37 °C for 30 min to allow for the cell sheet to adhere to the culture surface. Then a second cell sheet was placed on top of the first and attached by aspiration of the media. After incubation at 37 °C for 30 min, triple-layer constructs were finally created using the same procedures. Triple-layer cardiac cell sheets were overlaid on the vascular bed perfused within the bioreactor system. The second triple-layer cardiac cell sheets were overlaid on the first graft after cultivation for 3 days and then the whole construct was further perfused for an additional 3 days. Further multi-step layering was performed by the same procedure. Morphological analyses For cross-sectional observation, tissues were fixed in 4% paraformaldehyde and routinely processed into 7-μm-thick paraffin-embedded sections. HE staining and Azan staining was performed using conventional methods. For the detection of ECs, deparaffinized sections were incubated with both a 1:200 dilution of anti-GFP mouse monoclonal antibody (Life Technologies, Carlsbad, OR) and a 1:100 dilution of anti-CD31 rabbit polyclonal antibody (Life Technologies) overnight at 4 °C. For the detection of cardiomyocytes, sections were incubated with a 1:200 dilution of anti-sarcomeric α-actinin mouse monoclonal antibody (Sigma, St Louis, MO) for 2 h. For the detection of smooth muscle cells, sections were incubated with a 1/100 dilution of anti-calponin mouse monoclonal antibody (Acris Antibodies, Herford, Germany). Specimens were then treated with both a 1:200 dilution of Alexa-Fluor-488-conjugated anti-rabbit IgG antibodies (Life Technologies) and Alexa-Fluor-568 conjugated anti-mouse IgG antibodies (Life Technologies) for 2 h at room temperature. Cell nuclei were then counterstained by ProLong Gold antifade reagent with DAPI (Life Technologies) for 5 min. Sections were finally visualized using confocal laser-scanning microscopy (LSM 510 META; Carl Zeiss, Jena, Germany). Analyses of media supply dynamics and tissue survival A custom-made electron multiplying-CCD camera system and AquaCosmos 2.6 software (ImageEM, Hamamatsu Photonics, Shizuoka, Japan) were used for real-time bioluminescent imaging during the cultivation. Samples were placed into the light-tight chamber of the CCD camera system, and a grayscale surface image was taken under weak illumination. For the in vitro study, the cultivated tissue was continuously perfused with 0.1% D-luciferin firefly potassium salt (Promega, Madison, WI) at 50 μl min −1 in the bioreactor system. For the in vivo study, rats were anesthetized with 2% inhaled isoflurane, and 500 μl of 3.3% D -luciferin firefly potassium salt was injected into the superficial dorsal vein of the penis 2 min before imaging. The photon intensity of the cell sheet constructs was expressed as total flux, in units of photons per second. For anatomical localization, a pseudo colour image representing the light intensity (blue, least intense; red, most intense) was generated in Living Image and superimposed over the grayscale reference image. Image acquisition with two-photon laser-scanning microscopy The newly formed vessels were imaged using a two-photon laser-scanning microscopy system with FLUOVIEW version 3.1 software (FV1000MPE, Olympus, Tokyo, Japan) employing X25 objective lens (XLPLN25XWMP, numerical aperture=1.05, working distance=2.0 mm). The brightness compensation function in the z direction was used to change the detector sensitivity and laser power. The contribution of cocultured ECs was determined by detecting GFP signals from fluorescent images obtained after the constructs were finally perfused with 1% tetramethylrhodamine dextran (MW 2 million, Life Technologies) at 50 μl min −1 or 2% red fluorescent microspheres suspended in media (FluoSpheres, 4 μm in size, Life Technologies) at 50 μl min −1 . A series of X−Y images through the 3-D reconstruction data (500 × 500 × 200 μm volume) were obtained. Fabricated 3-D tissue transplantation to the neck To pursue the possibility of ectopic transplantation, separate F344 athymic rats (250–350 g, male, Charles River Japan) were anesthetized with 2% inhaled isoflurane and skin incisions were made in the neck to expose the underlying tissue. The common carotid artery and the jugular vein were exposed and isolated from their peripheries, and then clamped to prevent subsequent bleeding. The in vitro engineered constructs were connected to the neck vessels by a cuff technique as previously reported [17] . Briefly, the femoral artery and vein were introduced into 22 and 21-gauge cuffs, respectively, and were everted and secured with circumferential 6-0 silk sutures. The carotid artery and the jugular vein were gently slipped over the cuff that had been fixed to the femoral artery and vein, and secured again with circumferential 6-0 silk sutures. After the clamps were removed and the graft beating was confirmed, the incision was closed. After 2 weeks the survival of the graft was examined using the bioluminescent imaging system and then the rats were euthanized. Video capture Macroscopic images of pulsatile myocardial tissue grafts were recorded by a motion analysing microscope (VW5000, KEYENCE, Tokyo, Japan). The videos were edited with Adobe Premiere Pro 4.0 software. Data analysis All data are expressed as mean±s.d. An unpaired Student’s t -test was performed to compare the two groups. One-way analysis of variance was used for multiple group comparisons. If the F -distribution was significant, a Fisher’s LSD test was used to specify differences between groups. A P -value of <0.05 was considered significant. How to cite this article: Sekine, H. et al. In vitro fabrication of functional three-dimensional tissues with perfusable blood vessels. Nat. Commun. 4:1399 doi: 10.1038/ncomms2406 (2013).